Unfolded protein response, activated by OASIS family transcription factors, promotes astrocyte differentiation OASIS is a member of the CREB/ATF family of transcription factors and modulates cell- or tissue-specific unfolded protein response signalling. Here we show that this modulation has a critical role in the differentiation of neural precursor cells into astrocytes. Cerebral cortices of mice specifically deficient in OASIS ( Oasis −/− ) contain fewer astrocytes and more neural precursor cells than those of wild-type mice during embryonic development. Furthermore, astrocyte differentiation is delayed in primary cultured Oasis −/− neural precursor cells. The transcription factor Gcm1, which is necessary for astrocyte differentiation in Drosophila , is revealed to be a target of OASIS. Introduction of Gcm1 into Oasis −/− neural precursor cells improves the delayed differentiation of neural precursor cells into astrocytes by accelerating demethylation of the Gfap promoter. Gcm1 expression is temporally controlled by the unfolded protein response through interactions between OASIS family members during astrocyte differentiation. Taken together, our findings demonstrate a novel mechanism by which OASIS and its associated family members are modulated by the unfolded protein response to finely control astrocyte differentiation. To manage the burden of protein synthesis, cells augment the folding capacity of the endoplasmic reticulum (ER) in response to the accumulation of unfolded proteins. This is called the unfolded protein response (UPR) [1] , [2] . In mammalian cells, the three major transducers of the UPR are PKR-like endoplasmic reticulum kinase [3] , inositol-requiring 1 (refs 4 , 5 ), and activating transcription factor 6 (ATF6) [6] , [7] . Additionally, novel types of ER stress transducers that are structurally included in the CREB/ATF family and share a region of high sequence similarity with ATF6 have been identified [8] , [9] . These proteins have a transmembrane domain, which allows them to associate with the ER, a transcription-activation domain and a basic leucine zipper (bZIP) domain. These ER stress transducers include OASIS [10] , [11] , [12] , BBF2H7 [13] , [14] , CREBH [15] , [16] , CREB4 (refs 17 , 18 , 19 ), and Luman [20] , and are collectively referred to as OASIS family members. These molecules have unique cell- or tissue-specific expression patterns, indicating that OASIS family members may be associated with a distinct physiological response that is dependent on the cell or tissue. Oasis was originally identified as a gene that is specifically induced in long-term cultured astrocytes. Under normal conditions, OASIS is expressed at the ER membrane. In response to ER stress, OASIS is cleaved at the transmembrane region, and processed fragments of OASIS (the OASIS amino-terminus) containing the bZIP domain are translocated into the nucleus to promote transcription of target genes [10] , [11] , [12] . In vivo , OASIS is preferentially expressed in osteoblasts of bone tissues and astrocytes in the central nervous system (CNS). Oasis -deficient ( Oasis −/− ) mice exhibit severe osteopaenia caused by a decrease in the levels of type I collagen, a major component of the bone matrix and an OASIS target gene in osteoblasts [21] . In the CNS, OASIS is significantly induced in astrocytes after brain injury [10] . OASIS is also upregulated in reactive astrocytes after neuronal degeneration induced by kainic acid. The number of glial fibrillary acidic protein (GFAP)-positive reactive astrocytes was decreased in the hippocampi of Oasis −/− mice compared with those of wild-type (WT) mice [22] , indicating that the number of mature reactive astrocytes is decreased in Oasis −/− mice after brain injury. Although these findings suggest that OASIS is involved in the proliferation and differentiation of astrocytes, the functional details of OASIS in astrocytes remain unclear. The glial cell missing ( gcm ) gene was identified in Drosophila through the study of loss-of-function mutants [23] , [24] , [25] . Mutation in the gcm gene causes presumptive glial cells to differentiate into neurons, whereas ectopic expression of gcm makes all CNS cells differentiate into glial cells. Thus, gcm functions as a binary switch between glial and neuronal fates [26] . Two gcm homologues ( Gcm1 and Gcm2 ) have been identified in mice [27] . Gcm1 and Gcm2 encode transcription factors with a unique DNA-binding domain called the GCM-motif within their N-terminal regions allowing these factors to bind to GCM-binding sites [28] and regulate the expression of several genes [29] . The introduction of Gcm1 into cultured brain cells derived from mice resulted in the induction of an astrocyte lineage [30] . Recent work showed that mammalian Gcm1 and Gcm2 are involved in the genetic regulation of Hes5 transcription by accelerating DNA demethylation followed by induction of neural stem cells in the early embryonic stage [31] . However, the roles of Gcm in the differentiation of neural precursor cells (NPCs) into glial cell lineage in mammals are still unknown. Here we show that the UPR signalling mediated by OASIS and its associated family members, regulate the expression of Gcm1 and subsequently, differentiation of NPCs into astrocytes, via the demethylation of the Gfap promoter. Oasis −/− mice exhibit decrease in the number of astrocytes OASIS is structurally similar to an ER stress sensor ATF6, and contains a transmembrane domain, a transcription-activation domain and a bZIP domain at its N-terminus ( Fig. 1a ). To examine the expression of OASIS in the embryonic CNS, we performed in situ hybridization using mouse cerebral cortices. Although signals for Oasis messenger RNA were hardly observed in the cerebral cortices of embryonic day (E) 14.5 mice, strong signals were detected at E16.5 and E18.5 ( Fig. 1b ). Western blotting showed that both full-length and N-terminal OASIS (an active form) were expressed at E16.5 and the amounts of these proteins were increased at E18.5 ( Fig. 1c ), the findings of which are consistent with the findings regarding expression of Oasis mRNA. These data indicate that OASIS is expressed in the cerebral cortices of mouse embryos in the late stages of embryonic development. It is well known that astrocytes are largely differentiated from NPCs, around birth [32] . We noticed that upregulation of OASIS was synchronized with the initiation of differentiation of NPCs into astrocytes, and we hypothesized that OASIS may be involved in the regulation of astrocyte differentiation. To verify this hypothesis, we first investigated the expression of astrocyte and NPC markers in the embryonic stages by immunohistochemistry using cerebral cortices of WT and Oasis −/− mice. The numbers of cells positive for GFAP, an astrocyte marker, were significantly higher in the cerebral cortices of WT mice than in those of Oasis −/− mice from E16.5 ( Fig. 1d ). By contrast, those of nestin, an NPC marker, were higher in the cerebral cortices of Oasis −/− mice than in those of WT mice at E16.5 and E18.5 ( Fig. 1e ). The double staining of GFAP and OASIS ( Fig. 1f ), or GFAP and nestin ( Fig. 1g ), showed that GFAP and OASIS were co-expressed in the same cells, but not GFAP and nestin ( Fig. 1f,g ). To examine the expression levels of each marker, we carried out western blotting ( Fig. 1h ). In the embryonic stages, the expression levels of GFAP and S100β were markedly lower, and those of nestin and brain lipid-binding protein, NPC and radial glial cell markers, respectively, were higher in the cerebral cortices of Oasis −/− mice ( Fig. 1h,i ; Supplementary Fig. 1 ). These results suggest that differentiation of astrocytes from NPCs may be disturbed in the cerebral cortices of Oasis −/− mice in the embryonic stages. 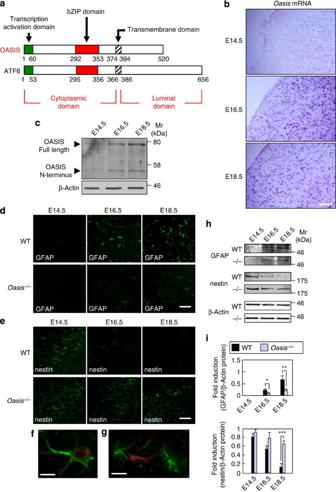Figure 1: Cerebral cortices ofOasis−/−mice. (a) Predicted peptide features of mouse OASIS and ATF6. (b)In situhybridization ofOasismRNA in the cerebral cortices of embryonic day (E) 14.5, E16.5 and E18.5 mice.Oasisexpression was induced in the cerebral cortices of E16.5 and E18.5 mice. Scale bar, 150 μm. (c) Western blotting of OASIS in the cerebral cortices of E14.5, E16.5 and E18.5 mice. Both full-length OASIS and its N-terminus were detected at E16.5 and were increased at E18.5. (d,e) Immunohistochemical analysis of (d) GFAP and (e) nestin in the cerebral cortices of E14.5, E16.5 and E18.5 WT andOasis−/−mice. InOasis−/−mice, the number of GFAP-positive cells was lower and that of nestin-positive cells was higher at E16.5 and E18.5 mice. Scale bars, 100 μm. (f,g) Double staining of GFAP (green) and OASIS (red) (f), GFAP (green) and nestin (red) (g) in the cerebral cortices of E18.5 WT mice. Scale bars, 50 μm. (h) Western blotting of GFAP and nestin in the cerebral cortices of WT andOasis−/−mice. (i) Quantitative analysis of protein expression levels in (h). All bars represent the mean values ±s.d. of three experiments. Significant difference was determined by unpaired Student's-t-test. *P<0.05, **P<0.01, ***P<0.001, between indicated pairs. Figure 1: Cerebral cortices of Oasis −/− mice. ( a ) Predicted peptide features of mouse OASIS and ATF6. ( b ) In situ hybridization of Oasis mRNA in the cerebral cortices of embryonic day (E) 14.5, E16.5 and E18.5 mice. Oasis expression was induced in the cerebral cortices of E16.5 and E18.5 mice. Scale bar, 150 μm. ( c ) Western blotting of OASIS in the cerebral cortices of E14.5, E16.5 and E18.5 mice. Both full-length OASIS and its N-terminus were detected at E16.5 and were increased at E18.5. ( d , e ) Immunohistochemical analysis of ( d ) GFAP and ( e ) nestin in the cerebral cortices of E14.5, E16.5 and E18.5 WT and Oasis −/− mice. In Oasis −/− mice, the number of GFAP-positive cells was lower and that of nestin-positive cells was higher at E16.5 and E18.5 mice. Scale bars, 100 μm. ( f , g ) Double staining of GFAP (green) and OASIS (red) ( f ), GFAP (green) and nestin (red) ( g ) in the cerebral cortices of E18.5 WT mice. Scale bars, 50 μm. ( h ) Western blotting of GFAP and nestin in the cerebral cortices of WT and Oasis −/− mice. ( i ) Quantitative analysis of protein expression levels in ( h ). All bars represent the mean values ±s.d. of three experiments. Significant difference was determined by unpaired Student's- t -test. * P <0.05, ** P <0.01, *** P <0.001, between indicated pairs. Full size image Differentiation of NPCs is inhibited in Oasis −/− NPCs Next, we investigated the expression of astrocyte and NPC markers using primary cultured NPCs prepared from E14.5 mice telencephalons. To promote differentiation of NPCs into astrocytes, the activation of Stat3 mediated by the stimulation of cytokines such as leukaemia inhibitory factor (LIF) is needed [32] , [33] , [34] , [35] , [36] . The bone morphogenetic protein (BMP) family is another group of astrocyte-inducing cytokines, members of which activate Smads [32] , [35] , [37] . Therefore, we treated NPCs with LIF and BMP2 (on day 0). During the differentiation of WT NPCs into astrocytes, the expression level of Gfap was increased, and conversely, that of Nestin was decreased ( Fig. 2a ). In Oasis −/− cells, the induction of Gfap expression and the reduction of Nestin expression were significantly impaired ( Fig. 2a ). The expression levels of these proteins coincided with those of their mRNAs ( Fig. 2b ). These results are consistent with in vivo findings that astrocyte differentiation is disturbed in Oasis −/− mice. Interestingly, when the culture was continued for a long time, the expression levels of these genes were not different between WT and Oasis −/− cells (data not shown). Thus, we concluded that the differentiation of NPCs into astrocytes was delayed in Oasis −/− cells, but was not completely inhibited. The expression of neuronal nuclear antigen (NeuN), a neuronal marker, and glutathione S -transferase-pi (GSTπ), an oligodendrocyte marker, were not affected in Oasis −/− mice ( Supplementary Fig. S2 ), indicating that differentiation of NPCs into neurons or oligodendrocytes was intact in Oasis −/− mice. 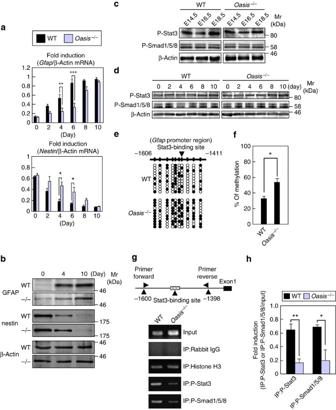Figure 2: Demethylation ofGfappromoter is inhibited in primary culturedOasis−/−NPCs. (a) RT–PCR analysis ofGfapandNestinin primary cultured NPCs treated with LIF and BMP2 for the indicated times. The upregulation ofGfapand the downregulation ofNestinwere inhibited inOasis−/−cells. (b) Western blotting of GFAP and nestin in primary cultured WT andOasis−/−NPCs treated with LIF and BMP2 for the indicated times. (c,d) Western blotting of phosphorylated (P)-Stat3 and P-Smad1/5/8 in the cerebral cortices of WT andOasis−/−mice (c) and primary cultured NPCs treated with LIF and BMP2 for the indicated times (d). The phosphorylation of these proteins was not affected byOasisdeficiency. (e) Bisulfite sequencing results for the CpG site within the Stat3 recognition sequence and other CpG sites around this sequence of theGfappromoter in NPCs treated with LIF and BMP2 for 4 days. (•) and (○) indicate methylated and demethylated CpG sites, respectively. Experiments were performed using 11 independent samples. (f) The percentages of methylated sites in theGfappromoter. (g) The top panel shows a schematic representation of theGfappromoter and the annealing sites of the primer set used in the ChIP assays. The bottom panel shows the results of PCR amplification of theGfappromoter region containing the Stat3-binding site (−1,398 to −1,600) after immunoprecipitation by indicated antibodies. Primary cultured NPCs treated with LIF and BMP2 for 4 days were used for ChIP assays. (h) Quantitative analysis of PCR amplification after immunoprecipitation by anti-P-Stat3 and anti-P-Smad1/5/8 antibodies in (g). All bars represent the mean values ±s.d. of 3 (a), 11 (f) and 4 (h) experiments. Significant difference was determined by unpaired Student's-t-test. *P<0.05, **P<0.01, ***P<0.001, between indicated pairs. Figure 2: Demethylation of Gfap promoter is inhibited in primary cultured Oasis −/− NPCs. ( a ) RT–PCR analysis of Gfap and Nestin in primary cultured NPCs treated with LIF and BMP2 for the indicated times. The upregulation of Gfap and the downregulation of Nestin were inhibited in Oasis −/− cells. ( b ) Western blotting of GFAP and nestin in primary cultured WT and Oasis −/− NPCs treated with LIF and BMP2 for the indicated times. ( c , d ) Western blotting of phosphorylated (P)-Stat3 and P-Smad1/5/8 in the cerebral cortices of WT and Oasis −/− mice ( c ) and primary cultured NPCs treated with LIF and BMP2 for the indicated times ( d ). The phosphorylation of these proteins was not affected by Oasis deficiency. ( e ) Bisulfite sequencing results for the CpG site within the Stat3 recognition sequence and other CpG sites around this sequence of the Gfap promoter in NPCs treated with LIF and BMP2 for 4 days. (•) and ( ○ ) indicate methylated and demethylated CpG sites, respectively. Experiments were performed using 11 independent samples. ( f ) The percentages of methylated sites in the Gfap promoter. ( g ) The top panel shows a schematic representation of the Gfap promoter and the annealing sites of the primer set used in the ChIP assays. The bottom panel shows the results of PCR amplification of the Gfap promoter region containing the Stat3-binding site (−1,398 to −1,600) after immunoprecipitation by indicated antibodies. Primary cultured NPCs treated with LIF and BMP2 for 4 days were used for ChIP assays. ( h ) Quantitative analysis of PCR amplification after immunoprecipitation by anti-P-Stat3 and anti-P-Smad1/5/8 antibodies in ( g ). All bars represent the mean values ±s.d. of 3 ( a ), 11 ( f ) and 4 ( h ) experiments. Significant difference was determined by unpaired Student's- t -test. * P <0.05, ** P <0.01, *** P <0.001, between indicated pairs. Full size image Demethylation of Gfap promoter is inhibited in Oasis −/− NPCs It is well known that the activation of Stat3 and Smads, and epigenetic regulation of the methylation status of the Gfap promoter are essential for differentiation of NPCs into astrocytes. Phosphorylated-Stat3 and Smads bind to demethylated sites in the Gfap promoter to form a Stat3-Smads-p300 complex and promote transcription of Gfap [32] , [35] , [37] , [38] . We examined levels of phosphorylated Stat3 and Smads and the methylation status of the Gfap promoter in Oasis −/− mice. Although the levels of phosphorylated Stat3 and Smads were not changed ( Fig. 2c,d ), the amount of demethylation of the Gfap promoter was significantly decreased in Oasis −/− NPCs (about 45% demethylated) compared with WT NPCs (about 65% demethylated) ( Fig. 2e,f ). Furthermore, the binding of Stat3 and Smads to the Gfap promoter was significantly inhibited in Oasis −/− NPCs ( Fig. 2g,h ). These findings suggest that the delayed astrocyte differentiation in Oasis −/− cells is caused by inhibition of demethylation of the Gfap promoter. The target of OASIS in NPCs is Gcm1 Previously, it was reported that OASIS could activate the transcription of Gcm1 in trophoblasts [39] . The Gcm1 Drosophila orthologue, gcm , has been reported to control neuronal and glial fates [23] , [24] , [25] . Further, a recent study showed that Gcm1 is involved in the demethylation of promoter regions in specific genes [31] . Gcm1 might be one of the direct target genes of OASIS in NPCs, and it is possible that OASIS is involved in the regulation of astrocyte differentiation through the expression of Gcm1 followed by the demethylation of the Gfap promoter. Therefore, we examined the expression levels of Gcm1 during astrocyte differentiation using primary cultured NPCs. Gcm1 was transiently upregulated during the differentiation of NPCs into astrocytes, and the expression pattern was similar to that of OASIS ( Fig. 3a,b ). However, Gcm1 was dramatically downregulated to about 50% of the WT level on day 4 in Oasis −/− cells. We infected primary cultured Oasis −/− NPCs with adenovirus expressing the OASIS N-terminus. Gcm1 expression was markedly upregulated by overexpression of the OASIS N-terminus ( Fig. 3c ). As OASIS is cleaved in response to ER stress, Gcm1 could be induced in NPCs exposed to ER stress, if Gcm1 is a direct target of OASIS in NPCs. Indeed, the expression level of Gcm1 was upregulated in WT NPCs under the ER stress condition. By contrast, the upregulation of Gcm1 was significantly inhibited in Oasis −/− NPCs ( Fig. 3d ). In the cerebral cortices of Oasis −/− mice, Gcm1 expression was downregulated ( Supplementary Fig. S3 ); the findings were consistent with the findings in primary cultured NPCs. 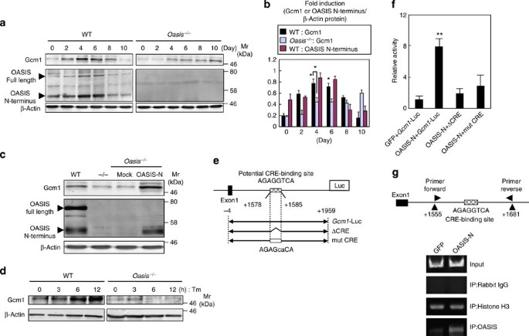Figure 3: Gcm1 is a direct target of OASIS in NPCs. (a) Western blotting of Gcm1 in NPCs treated with LIF and BMP2 for the indicated times. In WT cells, Gcm1 is transiently upregulated at the same time as OASIS. By contrast, it was significantly downregulated inOasis−/−NPCs. (b) Quantitative analysis of expression of Gcm1 and OASIS N-terminus in (a). (c) Western blotting of Gcm1 using NPCs cultured for 4 days. Adenoviruses expressing OASIS N-terminus were infected withOasis−/−NPCs. Mock indicates empty vector. (d) Western blotting of Gcm1 using NPCs treated with LIF and BMP2 for 4 days. Cells were exposed to 3 μg ml−1tunicamycin (Tm; an ER stressor) for the indicated times. (e) Scheme of the mouseGcm1promoter region and reporter constructs. TheGcm1-Luc construct consists of 2.0 kb from theGcm1promoter region. ΔCRE lacks the CRE-binding site (AGAGGTCA), and mut CRE is mutated (small letters of CRE sequence) in the CRE-binding site. Luc, luciferase gene. (f) Reporter assays using NPCs. Vectors expressing the mouse OASIS N-terminus or green fluorescent protein (GFP) were co-transfected with each reporter construct. GFP was used as a control. (g) The top panel shows a schematic representation of theGcm1promoter and the annealing sites of the primer set used in the ChIP assays. The bottom panel shows the results of PCR amplification of theGcm1promoter region containing the CRE-binding site (+1,555 to +1,681). NPCs were transfected with the vector expressing the mouse OASIS N-terminus. GFP was used as a control. All bars represent the mean values ±s.d. of three experiments. Significant difference between two samples was determined by unpaired Student'st-test (b). *P<0.05, between indicated pairs. Multiple comparisons were made using One way ANOVA followed by Tukey'spost hoctest. *P<0.05, **P<0.01, among WT cells (b) and all indicated samples (f). Figure 3: Gcm1 is a direct target of OASIS in NPCs. ( a ) Western blotting of Gcm1 in NPCs treated with LIF and BMP2 for the indicated times. In WT cells, Gcm1 is transiently upregulated at the same time as OASIS. By contrast, it was significantly downregulated in Oasis −/− NPCs. ( b ) Quantitative analysis of expression of Gcm1 and OASIS N-terminus in ( a ). ( c ) Western blotting of Gcm1 using NPCs cultured for 4 days. Adenoviruses expressing OASIS N-terminus were infected with Oasis −/− NPCs. Mock indicates empty vector. ( d ) Western blotting of Gcm1 using NPCs treated with LIF and BMP2 for 4 days. Cells were exposed to 3 μg ml −1 tunicamycin (Tm; an ER stressor) for the indicated times. ( e ) Scheme of the mouse Gcm1 promoter region and reporter constructs. The Gcm1 -Luc construct consists of 2.0 kb from the Gcm1 promoter region. ΔCRE lacks the CRE-binding site (AGAGGTCA), and mut CRE is mutated (small letters of CRE sequence) in the CRE-binding site. Luc, luciferase gene. ( f ) Reporter assays using NPCs. Vectors expressing the mouse OASIS N-terminus or green fluorescent protein (GFP) were co-transfected with each reporter construct. GFP was used as a control. ( g ) The top panel shows a schematic representation of the Gcm1 promoter and the annealing sites of the primer set used in the ChIP assays. The bottom panel shows the results of PCR amplification of the Gcm1 promoter region containing the CRE-binding site (+1,555 to +1,681). NPCs were transfected with the vector expressing the mouse OASIS N-terminus. GFP was used as a control. All bars represent the mean values ±s.d. of three experiments. Significant difference between two samples was determined by unpaired Student's t -test ( b ). * P <0.05, between indicated pairs. Multiple comparisons were made using One way ANOVA followed by Tukey's post hoc test. * P <0.05, ** P <0.01, among WT cells ( b ) and all indicated samples ( f ). Full size image To determine whether OASIS acts on the Gcm1 promoter and activates transcription of Gcm1 in NPCs, we performed promoter assays using a reporter gene carrying a 2.0-kb promoter region of Gcm1 ( Gcm1 -Luc) ( Fig. 3e ). In NPCs transfected with a Gcm1 -Luc construct, reporter activities were dramatically induced by expression of the OASIS N-terminus ( Fig. 3f ). The Gcm1 promoter includes a cAMP-responsive element (CRE) (+1,585 to +1,592 bp) that OASIS can bind to [10] . We next performed a promoter assay using the reporter constructs ΔCRE, which lacks the CRE-binding site, and mut CRE, which has a mutated CRE-binding site ( Fig. 3e ). In NPCs transfected with these constructs, reporter activities were markedly reduced, despite expression of the OASIS N-terminus ( Fig. 3f ). Furthermore, we performed chromatin immunoprecipitation (ChIP) assays and detected a high level of OASIS binding to the endogenous Gcm1 promoter in primary cultured NPCs transfected with the OASIS N-terminus ( Fig. 3g ). These results indicate that OASIS directly acts on the CRE sequence within the Gcm1 promoter and facilitates its transcription in NPCs. Mild ER stress and activation of UPR As shown in Fig. 3a , the levels of full-length OASIS and its N-terminus were increased during astrocyte differentiation. The OASIS N-terminus is produced by the cleavage of full-length OASIS in response to ER stress. It is possible that ER stress occurs during differentiation of NPCs into astrocytes. Therefore, we examined the expression of ER stress-related genes during astrocyte differentiation. Bip , p58 IPK and Erdj4 were slightly upregulated from day 2 to 6 during differentiation of WT and Oasis −/− NPCs into astrocytes ( Fig. 4a; Supplementary Fig. S4 ), indicating that all of signalling pathways from the major three sensors including PKR-like endoplasmic reticulum kinase, ATF6 and inositol-requiring 1, are activated during astrocyte differentiation. Furthermore, the transient upregulation of these genes was synchronized with the expression of the OASIS N-terminus ( Fig. 5d ), indicating that mild ER stress is transiently induced and that OASIS is activated by this mild ER stress during astrocyte differentiation. Although it is unknown, the roles of each pathway of major ER stress sensors. Next, we examined the roles of mild ER stress in cell fates including differentiation and cell death. To determine the level of ER stress during astrocyte differentiation, we quantified the expression levels of Erdj4 in NPCs exposed to several doses of dithiothreitol (DTT) or tunicamycin (Tm) ( Fig. 4b,c ). Consequently, we found that the level of ER stress in NPCs exposed to 125 μM DTT or 90 ng ml −1 Tm for 48 h was equal to that during astrocyte differentiation ( Fig. 4b,c ). This level of ER stress did not induce cell death ( Fig. 4d–f ), but activated UPR signalling pathways including the OASIS-Gcm1 pathway and promoted astrocyte differentiation after treatment with LIF and BMP2 ( Fig. 4g ). These results indicate that mild ER stress to a lesser extent than the levels that induce cell death is necessary for astrocyte differentiation. 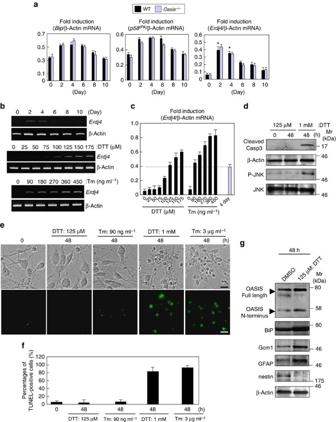Figure 4: Mild ER stress promotes astrocyte differentiation. (a) Real-time PCR analysis of ER stress-related genes in NPCs treated with LIF and BMP2 for the indicated times. Mild ER stress transiently occurred (from day 2 to day 6) during the differentiation of NPCs into astrocytes. (b) RT–PCR analysis ofErdj4in NPCs treated with LIF and BMP2 for the indicated times (top panel). Middle and bottom panels show the expression ofErdj4in NPCs exposed to DTT (an ER stressor) or Tm for 48 h. (c) Quantitative analysis of the expression ofErdj4in (b). The expression level ofErdj4in NPCs treated with LIF and BMP2 for 4 days was very similar to the expression levels in NPCs exposed to 125 μM DTT or 90 ng ml−1Tm for 48 h. The dotted line indicates the expression level ofErdj4in NPCs treated with LIF and BMP2 for 4 days. (d) Western blotting of cleaved caspase 3 (Casp3) and phosphorylated (P)-JNK in NPCs treated with LIF and BMP2 for 4 days. Cleaved Casp3 and P-JNK were not induced by the same level of mild ER stress observed during astrocyte differentiation. (e) Phase contrast images (top panels) and TUNEL staining (bottom panels) in NPCs treated with LIF and BMP2 for 4 days. Cell death was not induced by mild ER stress (125 μM DTT, 90 ng ml−1Tm). Scale bars, 25 μm. (f) The percentages of TUNEL-positive cells in (e). The number of TUNEL-positive cells was measured in five fields per well. (g) Western blotting of OASIS, BiP, Gcm1, GFAP and nestin in NPCs treated with LIF and BMP2 for 4 days. Mild ER stress activated UPR signalling and promoted astrocyte differentiation after treatment with LIF and BMP2. All bars represent the mean values ±s.d. of 4 (a,c) and 2 (f) experiments. Significant difference was determined by One-way ANOVA followed by Tukey'spost hoctest. *P<0.05, among WT cells. Figure 4: Mild ER stress promotes astrocyte differentiation. ( a ) Real-time PCR analysis of ER stress-related genes in NPCs treated with LIF and BMP2 for the indicated times. Mild ER stress transiently occurred (from day 2 to day 6) during the differentiation of NPCs into astrocytes. ( b ) RT–PCR analysis of Erdj4 in NPCs treated with LIF and BMP2 for the indicated times (top panel). Middle and bottom panels show the expression of Erdj4 in NPCs exposed to DTT (an ER stressor) or Tm for 48 h. ( c ) Quantitative analysis of the expression of Erdj4 in ( b ). The expression level of Erdj4 in NPCs treated with LIF and BMP2 for 4 days was very similar to the expression levels in NPCs exposed to 125 μM DTT or 90 ng ml −1 Tm for 48 h. The dotted line indicates the expression level of Erdj4 in NPCs treated with LIF and BMP2 for 4 days. ( d ) Western blotting of cleaved caspase 3 (Casp3) and phosphorylated (P)-JNK in NPCs treated with LIF and BMP2 for 4 days. Cleaved Casp3 and P-JNK were not induced by the same level of mild ER stress observed during astrocyte differentiation. ( e ) Phase contrast images (top panels) and TUNEL staining (bottom panels) in NPCs treated with LIF and BMP2 for 4 days. Cell death was not induced by mild ER stress (125 μM DTT, 90 ng ml −1 Tm). Scale bars, 25 μm. ( f ) The percentages of TUNEL-positive cells in ( e ). The number of TUNEL-positive cells was measured in five fields per well. ( g ) Western blotting of OASIS, BiP, Gcm1, GFAP and nestin in NPCs treated with LIF and BMP2 for 4 days. Mild ER stress activated UPR signalling and promoted astrocyte differentiation after treatment with LIF and BMP2. All bars represent the mean values ±s.d. of 4 ( a , c ) and 2 ( f ) experiments. Significant difference was determined by One-way ANOVA followed by Tukey's post hoc test. * P <0.05, among WT cells. 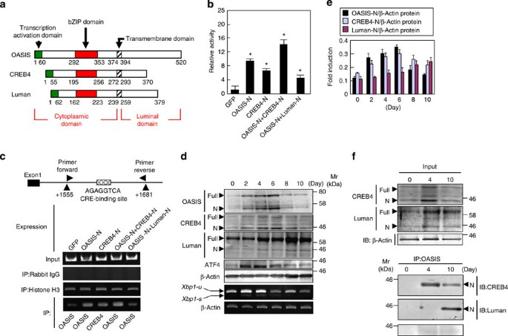Figure 5: OASIS and CREB4 form a heterodimer and promote Gcm1 expression. (a) Predicted peptide features of mouse OASIS, CREB4 and Luman. (b) Reporter assays in NPCs. Expression vectors for the N-terminus of mouse OASIS, CREB4, Luman and GFP were co-transfected withGcm1-Luc. GFP was used as a control. (c) The top panel shows a schematic representation of theGcm1promoter and the annealing sites of the primer set used in the ChIP assays. The bottom panel shows the results of PCR amplification of theGcm1promoter region containing the CRE-binding site (+1,555 to +1,681) after immunoprecipitation with indicated antibodies. NPCs were transfected with the expression vectors for the N-terminus of mouse OASIS, CREB4, Luman and GFP. GFP was used as a control. (d) Western blotting (OASIS, CREB4, Luman and ATF4) and RT–PCR (Xbp1) analysis in NPCs treated with LIF and BMP2 for the indicated times. Both full-length OASIS and CREB4 and their N-termini were upregulated from day 2 to 6 after treatment of NPCs with LIF and BMP2, synchronizing with the transient upregulation of ATF4 and spliced form ofXbp1(Xbp1-s). Luman N-terminus was upregulated after day 8 in these cells.Xbp-1-u: unspliced form ofXbp1. (e) Quantitative analysis of the expression of N-terminus of OASIS, CREB4 and Luman in (d). (f) Immunoprecipitation by anti-OASIS antibody followed by western blotting with the indicated antibodies using NPCs treated with LIF and BMP2 for the indicated times. OASIS N-terminus was robustly bound to CREB4 N-terminus on day 4. OASIS, and Luman N-terminus formed a complex on day 10. Input indicates cell lysates before immunoprecipitation. Full, Full length; N, N-terminus; IP, immunoprecipitation; IB, immunoblotting. All bars represent the mean values ±s.d. of three experiments. Significant difference was determined by One-way ANOVA followed by Tukey'spost hoctest. *P<0.05, among all indicated samples (OASIS-N, CREB4-N and OASIS-N+CREB4-N) or the samples named OASIS-N, OASIS-N+CREB4-N and OASIS-N+Luman-N (OASIS-N+Luman-N). Full size image Figure 5: OASIS and CREB4 form a heterodimer and promote Gcm1 expression. ( a ) Predicted peptide features of mouse OASIS, CREB4 and Luman. ( b ) Reporter assays in NPCs. Expression vectors for the N-terminus of mouse OASIS, CREB4, Luman and GFP were co-transfected with Gcm1 -Luc. GFP was used as a control. ( c ) The top panel shows a schematic representation of the Gcm1 promoter and the annealing sites of the primer set used in the ChIP assays. The bottom panel shows the results of PCR amplification of the Gcm1 promoter region containing the CRE-binding site (+1,555 to +1,681) after immunoprecipitation with indicated antibodies. NPCs were transfected with the expression vectors for the N-terminus of mouse OASIS, CREB4, Luman and GFP. GFP was used as a control. ( d ) Western blotting (OASIS, CREB4, Luman and ATF4) and RT–PCR ( Xbp1 ) analysis in NPCs treated with LIF and BMP2 for the indicated times. Both full-length OASIS and CREB4 and their N-termini were upregulated from day 2 to 6 after treatment of NPCs with LIF and BMP2, synchronizing with the transient upregulation of ATF4 and spliced form of Xbp1 ( Xbp1-s ). Luman N-terminus was upregulated after day 8 in these cells. Xbp-1-u : unspliced form of Xbp1 . ( e ) Quantitative analysis of the expression of N-terminus of OASIS, CREB4 and Luman in ( d ). ( f ) Immunoprecipitation by anti-OASIS antibody followed by western blotting with the indicated antibodies using NPCs treated with LIF and BMP2 for the indicated times. OASIS N-terminus was robustly bound to CREB4 N-terminus on day 4. OASIS, and Luman N-terminus formed a complex on day 10. Input indicates cell lysates before immunoprecipitation. Full, Full length; N, N-terminus; IP, immunoprecipitation; IB, immunoblotting. All bars represent the mean values ±s.d. of three experiments. Significant difference was determined by One-way ANOVA followed by Tukey's post hoc test. * P <0.05, among all indicated samples (OASIS-N, CREB4-N and OASIS-N+CREB4-N) or the samples named OASIS-N, OASIS-N+CREB4-N and OASIS-N+Luman-N (OASIS-N+Luman-N). Full size image Gcm1 expression modulation by OASIS family members ER stress-related CREB/ATF family members have the potential to bind to a CRE-binding site in promoter region and promote its transcription [13] , [16] , [40] . Thus, we checked the effects of CREB/ATF family members, including OASIS family members, on a Gcm1 -Luc reporter. Consequently, we found that CREB4 ( Fig. 5a ) promotes Gcm1 reporter activities ( Fig. 5b ; Supplementary Fig. S5 ). Furthermore, we detected the binding of CREB4 to endogenous Gcm1 promoter ( Fig. 5c ). Thus, not only OASIS but also CREB4 could activate the transcription of Gcm1 . Two previous reports showed that CREB4 does not bind to the CRE sequence (TGACGTCA) [18] , [19] . Thus far, CREB/ATF family members are known to bind to the several sequences such as TGACCTCA, TGAGGTCA, TGCCGTCA and TGAAGTCA [41] , [42] , [43] , [44] . AGAGGTCA sequence in the Gcm1 promoter region is not identical to TGACGTCA, which is the most common sequence as CREB/ATF family binding sequence. Therefore, it is possible that the manners of binding of OASIS and CREB4 are different from those of the other CREB/ATF family members. CREB/ATF family members are well known to form homodimers or heterodimers to promote transcription [16] , [45] . Thus, we examined the synergistic effects of CREB/ATF family members on Gcm1 promoter activities. In NPCs transfected with a Gcm1 -Luc construct, reporter activities were dramatically induced by co-expression of OASIS and CREB4 ( Fig. 5b ), and at the same time, the binding of OASIS to Gcm1 promoter was also significantly increased ( Fig. 5c ). Conversely, co-expression of OASIS and Luman, which is also an OASIS family member, resulted in significant downregulation of reporter activities and decreased binding of OASIS to the Gcm1 promoter ( Fig. 5b,c ). We next investigated endogenous expression of and direct interactions among OASIS family members during astrocyte differentiation. Both full-length OASIS and CREB4 and their N-termini were upregulated from day 2 to 6 after treatment of NPCs with LIF and BMP2 ( Fig. 5d,e ). Further, robust binding of OASIS N-terminus and CREB4 N-terminus was detected on day 4 ( Fig. 5f ). By contrast, binding of OASIS N-terminus and Luman N-terminus was observed on day 10 ( Fig. 5f ), suggesting that OASIS and CREB4 form a heterodimer in the early stage of astrocyte differentiation, and that Luman binds to OASIS in the late stage of astrocyte differentiation. Taken together, we concluded that an OASIS-CREB4 heterodimer activates transcription of Gcm1 during astrocyte differentiation. Conversely, Luman inhibits the formation of the OASIS-CREB4 heterodimer by binding to OASIS and downregulate the transcription of Gcm1 , followed by terminating differentiation of astrocytes. OASIS family members and Gcm1 promote astrocyte differentiation To examine whether OASIS family members and Gcm1 could rescue the delay in astrocyte differentiation observed in Oasis −/− NPCs, we introduced these molecules into primary cultured Oasis −/− NPCs. The expression levels of Gcm1 were upregulated by the introduction of the OASIS N-terminus, or co-expression of OASIS and CREB4 N-termini. However, introduction of the Luman N-terminus did not affect the expression of Gcm1 ( Fig. 6a ). Immunocytochemical analysis showed that the number of GFAP-positive cells was increased in NPCs treated with LIF and BMP2 for 4 days ( Fig. 6b ). Conversely, these cells were decreased in Oasis −/− NPCs or Oasis −/− NPCs expressing the empty vector ( Fig. 6c,d ). The decrease in the number of GFAP-positive Oasis −/− cells was restored to those of WT cells by introduction of OASIS N-terminus ( Fig. 6e,j ), CREB4 N-terminus ( Fig. 6f,j ) or Gcm1 ( Fig. 6g,j ). The co-expression of OASIS N-terminus and CREB4 N-terminus in Oasis −/− NPCs resulted in a greater improvement of the delay in astrocyte differentiation than did expression of OASIS N-terminus or CREB4 N-terminus alone ( Fig. 6 h,j ). The overexpression of Luman N-terminus in Oasis −/− NPCs could not restore the delay ( Fig. 6i,j ). These data indicate that OASIS-CREB4 heterodimerization followed by the induction of Gcm1 is necessary for accelerating astrocyte differentiation, and conversely, that Luman does not accelerate the differentiation of NPCs into astrocytes. 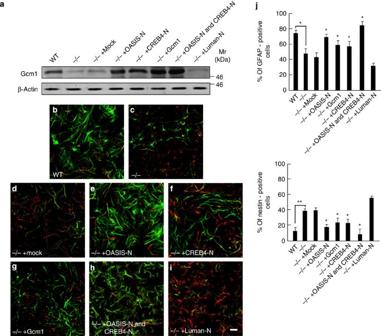Figure 6: OASIS family members and Gcm1 rescue the delay in astrocyte differentiation inOasis−/−NPCs. (a) Western blotting of Gcm1 in NPCs treated with LIF and BMP2 for 4 days. InOasis−/−NPCs, Gcm1 was upregulated by the introduction of the OASIS N-terminus, the CREB4 N-terminus, or co-expression of both. However, expression of the Luman N-terminus did not affect the expression of Gcm1. Mock indicates empty vector. (b–i) Immunostaining of GFAP (green) and nestin (red) in primary cultured NPCs treated with LIF and BMP2 for four days. Mock indicates empty vector. Scale bar, 50 μm. (j) The percentages of GFAP- (left panel) and nestin-positive cells (right panel) in (b–i). The number of positive cells was measured in five fields per well. All bars represent the mean values ±s.d. of ten experiments. Significant difference between two samples was determined by unpaired Student'st-test. *P<0.05, **P<0.01, between indicated pairs. Multiple comparisons were made using One-way ANOVA followed by Tukey'spost hoctest. *P<0.05, among all indicated samples except for WT. Figure 6: OASIS family members and Gcm1 rescue the delay in astrocyte differentiation in Oasis −/− NPCs. ( a ) Western blotting of Gcm1 in NPCs treated with LIF and BMP2 for 4 days. In Oasis −/− NPCs, Gcm1 was upregulated by the introduction of the OASIS N-terminus, the CREB4 N-terminus, or co-expression of both. However, expression of the Luman N-terminus did not affect the expression of Gcm1. Mock indicates empty vector. ( b – i ) Immunostaining of GFAP (green) and nestin (red) in primary cultured NPCs treated with LIF and BMP2 for four days. Mock indicates empty vector. Scale bar, 50 μm. ( j ) The percentages of GFAP- (left panel) and nestin-positive cells (right panel) in ( b – i ). The number of positive cells was measured in five fields per well. All bars represent the mean values ±s.d. of ten experiments. Significant difference between two samples was determined by unpaired Student's t -test. * P <0.05, ** P <0.01, between indicated pairs. Multiple comparisons were made using One-way ANOVA followed by Tukey's post hoc test. * P <0.05, among all indicated samples except for WT. Full size image Gcm1 is involved in demethylation of Gfap promoter As shown in Fig. 2 , demethylation of Gfap promoter was inhibited in Oasis −/− NPCs. To examine the mechanisms responsible for the impaired methylation status of the Gfap promoter in Oasis −/− NPCs, we performed bisulfite sequencing using the Gfap promoter ( Fig. 7a,b ). In NPCs cultured for 4 days, demethylation in the control was suppressed by transfection with a Gcm1 -specific short interfering RNA (siRNA) ( Fig. 7a,b ). In Oasis −/− NPCs, demethylation of Gfap promoter was also inhibited. The introduction of OASIS N-terminus or Gcm1 into Oasis −/− NPCs resulted in restoration of the Gfap demethylation status ( Fig. 7a,b ). 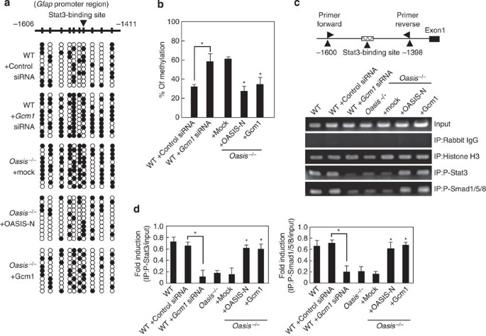Figure 7: Gcm1 is involved in demethylation of theGfappromoter. (a) Bisulfite sequencing results for theGfappromoter in primary cultured NPCs treated with LIF and BMP2 for four days. (•) and (○) indicate methylated and unmethylated CpG sites, respectively. Experiments were performed using 11 independent samples. Mock indicates empty vector. (b) The percentages of methylated sites in theGfappromoter. (c) The top panel shows a schematic representation of theGfappromoter and the annealing sites of the primer set used in the ChIP assays. The bottom panel shows the results of PCR amplification of theGfappromoter region containing the Stat3-binding site (−1,398 to −1,600) after immunoprecipitation with the indicated antibodies. Primary cultured NPCs treated with LIF and BMP2 for 4 days were used for ChIP assays. (d) Quantitative analysis of PCR amplification after immunoprecipitation by anti-P-Stat3 (top panel) and anti-P-Smad1/5/8 (bottom panel) antibodies in (c). All bars represent the mean values ±s.d. of 11 (b) and 4 (d) experiments. Significant difference between two samples was determined by unpaired Student'st-test. *P<0.05, between indicated pairs. Multiple comparisons were made using One-way ANOVA followed by Tukey'spost hoctest. *P<0.05, among the samples named +mock, +OASIS-N and +Gcm1 (b) andOasis−/−, +mock, +OASIS-N and +Gcm1 (d). Figure 7: Gcm1 is involved in demethylation of the Gfap promoter. ( a ) Bisulfite sequencing results for the Gfap promoter in primary cultured NPCs treated with LIF and BMP2 for four days. (•) and ( ○ ) indicate methylated and unmethylated CpG sites, respectively. Experiments were performed using 11 independent samples. Mock indicates empty vector. ( b ) The percentages of methylated sites in the Gfap promoter. ( c ) The top panel shows a schematic representation of the Gfap promoter and the annealing sites of the primer set used in the ChIP assays. The bottom panel shows the results of PCR amplification of the Gfap promoter region containing the Stat3-binding site (−1,398 to −1,600) after immunoprecipitation with the indicated antibodies. Primary cultured NPCs treated with LIF and BMP2 for 4 days were used for ChIP assays. ( d ) Quantitative analysis of PCR amplification after immunoprecipitation by anti-P-Stat3 (top panel) and anti-P-Smad1/5/8 (bottom panel) antibodies in ( c ). All bars represent the mean values ±s.d. of 11 ( b ) and 4 ( d ) experiments. Significant difference between two samples was determined by unpaired Student's t -test. * P <0.05, between indicated pairs. Multiple comparisons were made using One-way ANOVA followed by Tukey's post hoc test. * P <0.05, among the samples named +mock, +OASIS-N and +Gcm1 ( b ) and Oasis −/−, +mock, +OASIS-N and +Gcm1 ( d ). Full size image We further examined whether demethylation of Gfap promoter by OASIS-Gcm1 signalling induces binding of the Stat3-Smads-p300 complex to the promoter by performing ChIP assays using primary cultured NPCs ( Fig. 7c,d ). The binding of Stat3 and Smads to the endogenous Gfap promoter was inhibited in NPCs transfected with the Gcm1 -specific siRNA ( Fig. 7c,d ). In Oasis −/− NPCs, binding of Stat3 and Smads was also inhibited. The introduction of the OASIS N-terminus or Gcm1 into Oasis −/− NPCs restored the binding of Stat3 and Smads to the Gfap promoter to the levels seen in WT cells ( Fig. 7c,d ). These data suggest that the activation of OASIS-Gcm1 signalling accelerates demethylation of the Gfap promoter followed by binding of Stat3-Smads-p300 complex. It has been reported that the epigenetic regulation of the methylation status of the Gfap promoter is essential for accelerating differentiation of NPCs into astrocytes, and that the impairment of demethylation of the Gfap promoter disturbs astrocyte differentiation [38] . However, the regulatory mechanisms underlying demethylation of the Gfap promoter have remained unclear. In this study, we found that Gcm1, a direct target of OASIS, regulates the methylation status of the Gfap promoter followed by accelerating astrocyte differentiation. Interestingly, Gcm1 expression was fine-tuned by the dynamic interaction among OASIS family members that are activated by ER stress, during astrocyte differentiation. Thus, the spatio-temporal control of Gcm1 expression could contribute to production of functional and mature astrocytes. In this context, this report is the first to show that UPR signalling is linked to astrocyte differentiation. It is well known that not only epigenetic regulation but also the activation of Stat3 and Smads is essential for differentiation of NPCs into astrocytes [32] , [35] , [37] . However, the activation of these transcription factors was not affected in Oasis −/− mice ( Fig. 2c,d ). These findings strongly suggest that OASIS-Gcm1 signalling specially acts to regulate demethylation of the Gfap promoter, during astrocyte differentiation. We found that Gcm1 is a target gene of OASIS in the CNS. This conclusion is supported by the fact that (1) Gcm1 is significantly downregulated in the cerebral cortices and primary cultured NPCs of Oasis −/− mice; (2) a CRE-binding site that OASIS can bind to exist in the Gcm1 promoter region; (3) overexpression of the OASIS N-terminus upregulated Gcm1 promoter activities; (4) Gcm1 promoter activities were drastically decreased by mutation or deletion of the CRE-binding site; and (5) OASIS directly binds to the Gcm1 promoter. Gcm homologues have been shown to be involved as master regulators in key steps of differentiation processes [39] . In addition to astrocyte differentiation, Gcm1 is also essential for the differentiation of trophoblasts into syncytiotrophoblasts [39] . The promoter region of Gcm1 contains several CRE-binding sites containing the OASIS-binding site, we showed in this study. The effects of various CREB/ATF transcription factors on the Gcm1 promoter should be precisely analysed to elucidate the detailed mechanisms underlying cell differentiation regulated by Gcm1. The mammalian homologues of gcm are Gcm1 and Gcm2 . These molecules show little homology and have no common functional domains except for the GCM-motif [28] . Previous data have shown that both have the potential to accelerate demethylation of the Hes5 promoter by direct binding to the GCM-binding site in the promoter followed by acquiring the stem cell properties, but Gcm2 is a more crucial factor than Gcm1 for the demethylation of the Hes5 promoter because of the lower expression of Hes5 in Gcm2 −/− mice than in Gcm1 −/− mice [31] . In our data, expression of Gcm2 was not changed in Oasis −/− mice (data not shown), indicating that Gcm2 is not associated with the impaired differentiation of astrocytes observed in Oasis −/− mice. The expression of Gcm1 was significantly upregulated in the late stage of mouse embryonic development ( Supplementary Fig. S3 ), whereas that of Gcm2 was transiently upregulated in the early stage [31] . Therefore, we presume that Gcm2 is mainly involved in the demethylation of Hes5 promoter in the early stage of mouse embryonic development, and conversely, that Gcm1 mainly has a role in the demethylation of the Gfap promoter in the late stage. The distinct expression patterns and target promoters for demethylation between Gcm1 and Gcm2 may determine glial and neuronal cell lineages, respectively. We showed that OASIS, CREB4 and Luman activate the UPR signalling in response to mild ER stress, during astrocyte differentiation. Previous studies have shown that UPR signalling activated by mild ER stress is crucial for the differentiation of secretory cells including osteoblasts [21] , [46] , [47] , [48] , chondrocytes [14] and plasma cells [49] . During the differentiation of progenitor cells into these mature secretory cells, secretory materials are gradually produced, and abundant nascent proteins are delivered to the ER. Such an event may serve as a trigger for mild ER stress. Astrocytes also synthesize and secrete various neurotrophic factors and cytokines. During differentiation of NPCs into mature astrocytes, UPR signalling in response to the mild ER stress caused by production of abundant secretory proteins could be activated. Indeed, we found that ER stress-related genes were transiently upregulated during astrocyte differentiation. However, it remains unclear what extent of ER stress is needed for cell differentiation or how such mild ER stress activates only UPR signalling, but does not cause ER stress-induced apoptosis. The cerebral cortices of Oasis −/− mice contained few astrocytes in the embryonic stages, but interestingly, the numbers of astrocytes completely recovered to those in WT mice in adulthood (data not shown). We showed that transfection of NPCs with the CREB4 N-terminus activated the transcription of Gcm1 . Although the detailed underlying mechanisms are unknown, it is possible that CREB4 has the functional complement to promote astrocyte differentiation in Oasis −/− mice in adulthood. It has been reported that one of the aetiologies of psychiatric diseases such as schizophrenia and Rett syndrome is disturbance of the neuronal network caused by a decrease in the number of astrocytes in embryonic and infant stages [50] , [51] . Although the numbers of astrocytes in the cerebral cortices of Oasis −/− mice are normal in adulthood at first glance, a functional disturbance of the CNS may occur in adult Oasis −/− mice like in the CNS of such human diseases. It is necessary to perform advanced studies such as precise histological analysis and behavioural tests to clarify the association between OASIS and neuronal diseases. Mice C57BL/6 mice or Oasis −/− mice were used in this study. The Oasis −/− mice were previously established in our laboratory [21] . In all studies comparing WT and Oasis −/− mice, sex-matched littermates derived from the mating of Oasis +/– mice were used. The experimental procedures and housing conditions for animals were approved by the Committee of Animal Experimentation, Hiroshima University. Cell culture, plasmids, transfection and adenovirus Primary cultured NPCs were cultured as previously described [52] . Briefly, the telencephalons of E14.5 WT and Oasis −/− mice were triturated in Hank's balanced salt solution (Invitrogen) by mild pipetting with 1 ml pipette tips (Gilson, Greiner Bio-one). Dissociated cells were cultured in 1.27 g l −1 NaHCO3, 25 mg l −1 insulin (Sigma), 100 mg l −1 apo-transferrin (Sigma), 16 mg l −1 putrescin (Sigma), 30 nM sodium selenite (Sigma), 20 nM progesterone (Sigma) in D-MEM-F12 (Gibco), containing 10 ng ml −1 basic fibroblast growth factor (Pepro Tech) on culture dishes precoated with poly-ornithine (Sigma) and fibronectin (Sigma) for 4 days. The following day, the cells were stimulated with 50 ng ml −1 LIF (Sigma) and 50 ng ml −1 BMP2 (Sigma) to initiate astrocyte differentiation. For knockdown of Gcm1 , NPCs were transfected with a Gcm1-targeting siRNA (Ambion; 4390771) or a non-targeting siRNA (Thermo Scientific; D-001206-13-05) as a control using Lipofectamine 2000 reagent (Invitrogen). Complementary DNAs encoding the N-termini of mouse OASIS, BBF2H7, ATF6, Luman, CREBH and CREB4, the spliced form of XBP1, and full-length ATF4 were inserted into pCDNA3.1+ (Invitrogen). The complementary DNA sequences are summarized in Supplementary Table S1 . Cells were transfected with each expression plasmid using Lipofectamine 2000 reagent. The recombinant adenovirus carrying mouse OASIS was generated previously [21] . Adenovirus vectors expressing the mouse Gcm1 were constructed using the AdenoX Expression system (Clontech), according to the manufacturer's protocol. Immunohistochemistry Cerebral cortices of WT and Oasis −/− mice at the indicated stages were fixed in 4% paraformaldehyde (PFA). Samples were then dehydrated with ethanol, embedded in paraffin and sectioned (5 μm). Paraffin sections were stained with antibodies and visualized under a fluorescence microscope (BX51, Olympus) or a confocal microscope (FV1000D, Olympus). The following antibodies and dilutions were used: anti-GFAP (Sigma; 1:200), and anti-nestin (Abcam; 1:200). The anti-OASIS monoclonal antibody (1:500) was generated previously [21] . In situ hybridization In situ hybridization was performed using digoxigenin-labelled Oasis antisense RNA (cRNA) probes [21] . Oasis cRNA probes were made by in vitro transcription in the presence of digoxigenin-labelled dUTP, using Oasis cRNA subcloned into the pGEM-Teasy vector (Promega) as templates. Cerebral cortices were frozen immediately and sectioned (5 μm). Frozen sections were fixed for 20 min with 4% formalin. Then the sections were treated with 0.1% proteinase K for 5 min. After washing with PBS, the sections were re-fixed for 20 min with 4% formalin, and treated with 0.1 M triethanolamine, 2.5% anhydrous acetic acid for 10 min. Sections were prehybridized for 1 h at 37 °C in hybridization buffer (0.01% dextran sulfate, 0.01 M Tris–HCl pH 8.0, 0.05 M NaCl, 50% formamide, 0.2% sarcosyl, 1× Denhardt's solution, 0.5 mg ml −1 yeast tRNA, 0.2 mg ml −1 salmon testis DNA), and hybridized overnight at 55 °C. After washing with 4×saline sodium citrate buffer for 20 min at 60 °C followed by 2×saline sodium citrate buffer, 50% formamide for 30 min at 60 °C, sections were treated with RNaseA in RNase buffer (10 mM Tris–HCl pH 7.4, 1 mM 0.5 M EDTA (pH 8.0), 0.5 M NaCl) for 30 min at 37 °C to remove un-hybridized probe. After RNase treatment, sections were washed with 2×saline sodium citrate buffer, 50% formamide for 30 min at 60 °C, and then blocked with 1.5% blocking reagent in 100 mM Tris–HCl pH 7.5, 150 mM NaCl for 60 min at room temperature. For detection of digoxigenin-labelled cRNA probes, anti-digoxigenin antibody conjugated to alkaline phosphatase (Roche) was used at a dilution of 1:500, and colour was developed by incubation with 4-nitro blue tetrazolium chloride and 5-bromo-4-chloro-3-indolyl phosphate solution. Quantitative real-time PCR and RT–PCR Total RNA was isolated using an RNeasy kit (Qiagen) according to the manufacturer's protocol. First-strand cDNA was synthesized in a 20-μl reaction volume using random primers (Takara) and Moloney murine leukemia virus reverse transcriptase (Invitrogen). Quantitative real-time PCR reactions were performed using a Light Cycler 480 system II (Roche) and Light Cycler SYBR Green I Master (Roche). RT–PCR was performed using each specific primer set in a total volume of 30 μl containing 0.8 μM of each primer, 0.2 mM dNTPs, 3 units of Taq polymerase, and 10×PCR buffer (Agilent). The density of each band on RT–PCR was quantified using Photoshop Elements 2.0 (Adobe Systems). Primer sequences are summarized in Supplementary Table S2 . Western blotting Proteins were extracted from cells or mice cerebral cortices using cell extraction buffer containing 2.5 mM methionine, 33.3 mM Tris-acetate pH 8.5, 5 mM EDTA, 0.3% SDS, 1.5% Triton, and protease inhibitor cocktail (MBL). Lysates were incubated on ice for 45 min. After centrifugation at 15,000 g for 15 min, the soluble protein concentration was measured using BCA protein assay reagents (Pierce). The following antibodies and dilutions were used: anti-β-actin (Sigma; 1:3,000), anti-GFAP (Sigma; 1:1,000), anti-S100β (Abcam; 1:1,000), anti-nestin (Abcam; 1:500), anti-brain lipid-binding protein (Abcam; 1:500), anti-NeuN (CHEMICON; 1:1,000), anti-GSTπ (BD Transduction Laboratories; 1:1,000), anti-phosphorylated-Stat3 (Santa Cruz Biotechnology; 1:500), anti-phosphorylated-Smad1/5/8 (Cell Signaling; 1:1,000), anti-Gcm1 (Santa Cruz Biotechnology; 1:500), anti-Luman (Santa Cruz Biotechnology; 1:250), anti-ATF4 (Santa Cruz Biotechnology; 1:500), anti-ATF6 (Santa Cruz Biotechnology; 1:250), anti-JNK (Cell Signaling; 1:1,000), anti-phosphorylated-JNK (Cell Signaling; 1:1,000), anti-Caspase 3 (Cell Signaling; 1:1,000), anti-BiP (MBL; 1:1,000), and anti-XBP1 (Santa Cruz Biotechnology; 1:250). The anti-OASIS monoclonal antibody (1:1,000) was generated previously [21] . The anti-CREB4 polyclonal antibody (1:1,000) was generated by immunizing mice against mouse recombinant CREB4 (amino acids 1–162). The density of each band was quantified using Photoshop Elements 2.0 (Adobe Systems). Immunofluorescence Cells were fixed in 4% PFA and then permeabilized in 0.5% Triton-X 100. The following antibodies and dilutions were used: anti-GFAP (Sigma; 1:500), and anti-nestin (Abcam; 1:250). Cells were visualized under a fluorescence microscope or a confocal microscope (FV1000D, Olympus). The number of positive cells was measured in five fields per well. TUNEL assay Primary cultured NPCs prepared from E14.5 WT and Oasis −/− mice were fixed in 4% PFA and then permeabilized in 0.1% sodium citrate and 0.1% Triton-X 100. TdT-mediated dUTP nick end labeling (TUNEL) staining was performed using the Cell Death Detection kit, Fluorescein (Roche), according to the manufacturer's protocol. Cells were visualized under a fluorescence microscope. The number of positive cells was measured in five fields per well. Immunoprecipitation assay Cells were washed with PBS and lysed with 1 ml of 1% CHAPSO (Sigma) buffer. Cell lysates were centrifuged at 15,000 g at 4 °C for 15 min and supernatants collected and then incubated with anti-OASIS antibody overnight. Then, samples were incubated with protein G–Sepharose beads (GE Healthcare Life Sciences) for an additional 2 h at 4 °C. Beads were washed with TNE buffer, containing 10 mM Tris, 1 mM EDTA and 150 mM NaCl. Subsequently, samples were subjected to western blotting with anti-CREB4 or anti-Luman antibody. Luciferase assay Primary cultured NPCs prepared from E14.5 WT and Oasis −/− mice were cultured for 4 days and transfected with 0.2 μg of a pGL3 basic reporter plasmid carrying the firefly luciferase gene (Promega) and 0.02 μg of the reference plasmid pRL-SV40 carrying the Renilla luciferase gene under the control of the SV40 enhancer and promoter (Promega), together with 0.2 μg of an effector protein expression plasmid, using Lipofectamine 2000 reagent. UPRE-LUC reporter was kind gift from Ron Prywes (Columbia University) [53] . After 24 h, luciferase activities were measured using the Dual-Luciferase Reporter Assay System (Promega) and a luminometer (Berthold Technologies), according to the manufacturer's protocol. Relative activity was defined as the ratio of firefly luciferase activity to that of Renilla luciferase. Chromatin immunoprecipitation assay The chromatin immunoprecipitation assay was performed as previously described [10] . The primers used for the mouse Gcm1 promoter were: 5′-GAAAAATTATTAACATGTGTGAATGCAT-3′ (forward) and 5′-CTCAAAAGAGGGTGGTGGGGGGCTTA-3′ (reverse) yielding a 127-bp product. Those used for the mouse Gfap promoter were: 5′-CCTTCCCTATGGTGGGACTCATTAGGAG-3′ (forward) and 5′-CATGCTTGGGCTTCTGGTGTCTACTCCAG-3′ (reverse) yielding a 209-bp product. The following antibodies were used: anti-OASIS [21] , anti-CREB4 (generated by immunizing mice against mouse recombinant CREB4: amino acids 1–162), anti-histone H3 (Santa Cruz Biotechnology), and rabbit IgG (Sigma). Bisulfite sequencing Procedures were performed as previously described [52] . Sodium bisulfite treatment of genomic DNA was performed using a Methylamp DNA Modification kit (Epigentek), according to the manufacturer's protocol. The region in the Gfap promoter containing the Stat-binding site of the bisulfite-treated genomic DNA was amplified by PCR using the following primers: 5′-GGGATTTATTAGGAGAATTTTAGAAGTAG-3′ (forward) and 5′-TCTACCCATACTTAAACTTCTAATATCTAC-3′ (reverse). The PCR products were cloned into pCR–Blunt II-TOPO vector (Invitrogen) and at least 11 randomly selected clones were sequenced. Statistical analysis Statistical comparisons were made using the unpaired Student's- t -test (between two samples) and One-way ANOVA followed by Tukey's post hoc test (among multiple samples). The statistical significance of a difference between each sample was determined on the basis of a P -value <0.05. P -values of <0.05, 0.01 or 0.001 are described as * P <0.05, ** P <0.01, or *** P <0.001, respectively. How to cite this article: Saito, A. et al . Unfolded protein response, activated by OASIS family transcription factors, promotes astrocyte differentiation. Nat. Commun. 3:967 doi: 10.1038/ncomms1971 (2012).